Caspase-mediated activation ofCaenorhabditis elegansCED-8 promotes apoptosis and phosphatidylserine externalization During apoptosis, phosphatidylserine (PS), normally restricted to the inner leaflet of the plasma membrane, is exposed on the surface of apoptotic cells and serves as an ‘eat-me’ signal to trigger phagocytosis. It is poorly understood how PS exposure is activated in apoptotic cells. Here we report that CED-8, a Caenorhabditis elegans protein implicated in controlling the kinetics of apoptosis and a homologue of the XK family proteins, is a substrate of the CED-3 caspase. Cleavage of CED-8 by CED-3 activates its proapoptotic function and generates a carboxyl-terminal cleavage product, acCED-8, that promotes PS externalization in apoptotic cells and can induce ectopic PS exposure in living cells. Consistent with its role in promoting PS externalization in apoptotic cells, ced-8 is important for cell corpse engulfment in C. elegans . Our finding identifies a crucial link between caspase activation and PS externalization, which triggers phagocytosis of apoptotic cells. Phospholipids are major components of the plasma membrane and are asymmetrically distributed in the inner and outer leaflets of the plasma membrane, with phosphatidylcholine and sphingomyelin predominantly in the outer leaflet and phosphatidylserine (PS) and phosphatidylethanolamine in the inner leaflet of the plasma membrane [1] . During apoptosis, the asymmetrical distribution of phospholipids is disrupted, leading to the flipping of PS to the outer leaflet of the plasma membrane [2] , [3] . The externalized PS then serves as an ‘eat-me’ signal to trigger removal of apoptotic cells [4] . Caspases are a family of cysteine proteases that are activated during apoptosis to initiate multiple cell suicidal or disassembly events, including nuclear membrane breakdown, chromatin fragmentation and mitochondria elimination [5] . They promote cell death execution by cleaving and activating proapoptotic caspase substrates or inactivating anti-apoptotic caspase substrates [6] . How PS is externalized during apoptosis and whether caspases have a direct role in activating PS externalization are poorly understood and have been a long-standing issue in the field of apoptosis [4] , [7] . In the nematode Caenorhabditis elegans, the caspase-encoding gene ced-3 is required for the death of almost all cells programmed to die [8] , but how the CED-3 caspase kills the cell through cleavage of its downstream protein substrates remains largely unknown. DRP-1, a dynamin-related GTPase, and DCR-1, a ribonuclease important for small RNA biogenesis, have been identified as two important CED-3 substrates that are activated by CED-3 cleavage to promote mitochondrial elimination and to initiate chromosome fragmentation during apoptosis, respectively [9] , [10] . As in mammals, PS externalization occurs during C. elegans apoptosis [11] , [12] , [13] and is one of the earliest cell death events observed in worms [14] . In animals deficient in ced-3, few cells undergo apoptosis and PS is not externalized in cells that are programmed to die [11] , [14] . These observations suggest that CED-3 is required to activate the PS externalization process in apoptotic cells. The ced-8 gene was first identified as a gene important for controlling the kinetics of apoptosis in C. elegans [15] . In ced-8 loss-of-function ( lf ) mutants, the numbers of cell corpses in early embryonic stages are markedly reduced and more apoptotic cells appear in late embryonic stages and in the L1 larval stage, suggesting a delay of early embryonic cell deaths to later embryonic stages [15] . ced-8 encodes a protein with sequence similarity to the human XK membrane transporter [15] . Loss of human XK has been associated with the McLeod syndrome, a hereditary disease characterized by abnormalities in the neuromuscular and hematopoietic systems, including acanthocytic red blood cells, loss of erythrocyte Kx antigen and reduction of Kell antigens [16] , [17] , [18] . The mechanism by which ced-8 affects apoptosis is unknown, but genetic analysis suggests that it functions downstream of or in parallel to the C. elegans cell death inhibitor ced-9 (ref. 15 ). In this study, we present evidence that CED-8 is a substrate of the CED-3 caspase and acts downstream of CED-3 to promote cell killing. Cleavage of CED-8 by CED-3 generates an activated cleavage product, acCED-8, that is necessary and sufficient to mediate the proapoptotic functions of CED-8. Moreover, we find that CED-8 is important for PS externalization in apoptotic cells and phagocytosis and that acCED-8 can induce ectopic PS exposure in living cells. Our study thus identifies an important caspase mediator that activates PS externalization in response to caspase activation. CED-8 is a substrate of the CED-3 caspase In wild-type C. elegans embryos, most cell deaths occur during early embryogenesis (comma, 1.5-fold and 2-fold embryonic stages) and less cell deaths are seen during late embryogenesis (3-fold and 4-fold embryonic stages; Fig. 1a ). In a strong lf ced-8(n1891) mutant, the numbers of cell corpses in early embryonic stages are greatly reduced and significantly more apoptotic cells are found in late embryonic stages and in the L1 larval stage [15] , suggesting a delay of embryonic cell deaths ( Fig. 1a ). To understand how ced-8 acts to effect apoptosis, we first determined whether ced-8 acts downstream or upstream of the CED-3 caspase. We performed epistatic analysis of ced-8 and ced-3 using an integrated transgene ( smIs111 ) that expresses an activated form of CED-3 (acCED-3) under the control of the promoter of the C. elegans cell death initiator egl-1 (ref. 19 ). When smIs111 was placed in the ced-1(e1735); ced-3(n2433) mutant background, in which almost all naturally occurring cell deaths in C. elegans are blocked by a strong lf ced-3(n2433) mutation ( ced-1(e1735) blocks cell corpse engulfment and sensitizes quantification of apoptotic cells [20] ), acCED-3 still induced ectopic cell death and an average of 8 and 11 persistent cell corpses in 2-fold- and 4-fold-stage embryos, respectively ( Fig. 1b ). The ced-8(n1891) mutation significantly reduced the number of ectopic cell deaths induced by acCED-3 in ced-1(e1735) smIs111; ced-3(n2433) embryos ( Fig. 1b ), indicating that ced-8 probably acts downstream of ced-3 to promote apoptosis. 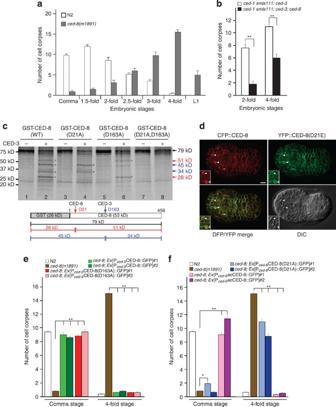Figure 1:ced-8acts downstream ofced-3and encodes a substrate of CED-3. (a) Appearance of apoptotic cell corpses in different stages of wild-type (N2) andced-8(n1891)embryos. (b)ced-8acts downstream ofced-3. Cell corpses were scored in 2-fold and 4-foldced-1(e1735) smIs111; ced-3(n2433)andced-1(e1735) smIs111; ced-3(n2433); ced-8(n1891)embryos. (c) Cleavage of CED-8 by CED-3in vitro. Top:35S-Met-labelled GST-CED-8 proteins (wild-type or mutants) were incubated with or without 5 ng purified CED-3 protease at 30 °C for 2 h and then resolved by 15% SDS–polyacrylamide gel electrophoresis. Bottom: a schematic diagram of GST-CED-8 and cleavage products generated by CED-3 (indicated by arrows). (d) Demonstration ofin vivocleavage of CED-8 by CED-3. CFP, YFP, CFP/YFP merged and differential contrast interference images of a comma-stageced-1(e1735)embryo expressing CFP::CED-8 and YFP::CED-8(D21E) are shown. CFP (pseudo-colour in red) is observed in the cytoplasm of apoptotic cells (arrowheads). YFP (pseudo-colour in green) remains localized to the plasma membrane. Scale bar, 5 μm. (e,f) Rescue of the delay-of-cell-death defect of theced-8(n1891)mutant by variousced-8transgenes. Cell corpses were scored in the following animals: (e) N2,ced-8(n1891), ced-8(n1891); ex[Pced-8CED-8::GFP] arrays #1–2 andced-8(n1891); ex[Pced-8CED-8(D163A)::GFP] arrays #1–2. (f) N2,ced-8(n1891), ced-8(n1891); ex[Pced-8CED-8(D21A)::GFP] arrays #1–2 andced-8(n1891); ex[Pced-8acCED-8::GFP] arrays #1–2. Comma- and 4-fold-stage transgenic embryos were examined. (a,b,e,f) They-axis represents average number of cell corpses scored and error bars represent s.e.m. (n=15). The significance of differences between results was determined by two-tailed Student’st-tests, *P<0.05; **P<0.001. Figure 1: ced-8 acts downstream of ced-3 and encodes a substrate of CED-3. ( a ) Appearance of apoptotic cell corpses in different stages of wild-type (N2) and ced-8(n1891) embryos. ( b ) ced-8 acts downstream of ced-3 . Cell corpses were scored in 2-fold and 4-fold ced-1(e1735) smIs111; ced-3(n2433) and ced-1(e1735) smIs111; ced-3(n2433); ced-8(n1891) embryos. ( c ) Cleavage of CED-8 by CED-3 in vitro . Top: 35 S -Met-labelled GST-CED-8 proteins (wild-type or mutants) were incubated with or without 5 ng purified CED-3 protease at 30 °C for 2 h and then resolved by 15% SDS–polyacrylamide gel electrophoresis. Bottom: a schematic diagram of GST-CED-8 and cleavage products generated by CED-3 (indicated by arrows). ( d ) Demonstration of in vivo cleavage of CED-8 by CED-3. CFP, YFP, CFP/YFP merged and differential contrast interference images of a comma-stage ced-1(e1735) embryo expressing CFP::CED-8 and YFP::CED-8(D21E) are shown. CFP (pseudo-colour in red) is observed in the cytoplasm of apoptotic cells (arrowheads). YFP (pseudo-colour in green) remains localized to the plasma membrane. Scale bar, 5 μm. ( e , f ) Rescue of the delay-of-cell-death defect of the ced-8(n1891) mutant by various ced-8 transgenes. Cell corpses were scored in the following animals: ( e ) N2, ced-8(n1891), ced-8(n1891); ex [P ced-8 CED-8::GFP] arrays #1–2 and ced-8(n1891); ex [P ced-8 CED-8(D163A)::GFP] arrays #1–2. ( f ) N2, ced-8(n1891), ced-8(n1891); ex [P ced-8 CED-8(D21A)::GFP] arrays #1–2 and ced-8(n1891); ex [P ced-8 acCED-8::GFP] arrays #1–2. Comma- and 4-fold-stage transgenic embryos were examined. ( a , b , e , f ) The y -axis represents average number of cell corpses scored and error bars represent s.e.m. ( n =15). The significance of differences between results was determined by two-tailed Student’s t -tests, * P <0.05; ** P <0.001. Full size image As effectors of apoptosis that act downstream of caspases are often substrates of caspases [6] , [9] , [10] , [21] , we tested whether CED-8 is a substrate of the CED-3 protease. A glutathione S -transferase CED-8 fusion (GST-CED-8) was synthesized and labelled with 35 S -methionine in rabbit reticulocyte lysate and incubated with purified CED-3 protease [22] . 35 S -Met-labelled GST-CED-8 was cleaved by CED-3, yielding multiple cleavage products of ~51, 45, 34 and 28 kD ( Fig. 1c , lanes 1 and 2). On the basis of the sizes of the cleavage products and the known consensus CED-3 cleavage sites, D/EXXD, in which X can be any amino acid [22] , we inferred the locations of two principle CED-3 cleavage sites: between Asp 21 and Ala 22 and between Asp 163 and Gly 164. The amino-acid sequences amino terminal to these two potential cleavage sites (P 4 to P 1 ; EQED and ENTD) are consistent with the consensus CED-3 cleavage sites. When Asp 21 of CED-8 was replaced by Ala and the resulting mutant protein, GST-CED-8(D21A) was examined in the CED-3 cleavage assay, the 51- and 28-kD cleavage products expected from CED-3 cleavage at CED-8 Asp 21 were lost ( Fig. 1c , lanes 3 and 4), confirming that CED-3 cleaves CED-8 at Asp 21. Similarly, substitution of CED-8 Asp 163 with Ala blocked the production of the 45- and 34-kD cleavage products expected from CED-3 cleavage at CED-8 Asp 163 ( Fig. 1c , lanes 5 and 6). Moreover, substitutions of both Asp 21 and Asp 163 with Ala prevented cleavage of CED-8 by CED-3 ( Fig. 1c , lanes 7 and 8), indicating that these are two major in vitro CED-3 cleavage sites. Analysis of the CED-8 protein sequence using the TOPCONS program (consensus prediction of membrane protein topology) yields uniformed predictions that residues 1–34 are inside the cell, whereas residues 145–218 are extracellular and correspond to the site of the extracellular disulphide linkage of XK to Kell [16] , [23] . Therefore, Asp 163 is unlikely accessible to CED-3 in vivo. We examined whether CED-8 is cleaved by CED-3 in cells undergoing apoptosis using a yellow fluorescent protein (YFP) and cyan fluorescent protein (CFP) dual reporter assay. We generated a CFP fusion to the N terminus of wild-type CED-8 (CFP::CED-8) and a YFP fusion to the N terminus of CED-8(D21E) [YFP::CED-8(D21E)], which is resistant to CED-3 cleavage because D21E blocks CED-3 cleavage of CED-8 as well as D21A ( Supplementary Fig. S1 ). Both fusion proteins were expressed in C. elegans under the control of the native ced-8 promoter. In living cells, both CFP::CED-8 and YFP::CED-8(D21E) displayed identical plasma membrane localization indistinguishable from that of CED-8::GFP (green fluorescent protein) reported previously ( Fig. 1d and Supplementary Fig. S2a,b ) [15] . In cells undergoing apoptosis (arrowheads, Fig. 1d ), CFP was observed instead in the cytoplasm, suggesting that following CED-3 cleavage CFP disassociated from CED-8 localized on the plasma membrane and diffused into the cytoplasm. In comparison, YFP remained associated with CED-8(D21E) and localized to the plasma membrane in these apoptotic cells ( Fig. 1d ), indicating that CED-3 cleaves CED-8 at Asp 21 in vivo . CED-8 cleavage by CED-3 is critical for apoptosis We next examined whether the two in vitro CED-3 cleavage sites in CED-8 are important for its proapoptotic function in vivo . We tested whether transgenes expressing wild type or mutant forms of CED-8::GFP fusions under the control of the ced-8 gene promoter can rescue the delay-of-cell-death defect of the ced-8(n1891) mutant at two signature embryonic stages, the early comma embryonic stage and the late 4-fold embryonic stage ( Fig. 1a ). Compared with wild-type embryos, which had an average of 9 cell corpses in the comma stage and few cell corpse in the 4-fold stage, ced-8(n1891) embryos had 1–2 cell corpses in the comma stage and an average of 15 cell corpses in the 4-fold embryonic stage ( Fig. 1a ) [15] . Transgenes expressing wild-type CED-8 [P ced-8 CED-8::GFP] or mutant CED-8(D163A) [P ced-8 CED-8(D163A)::GFP] fully rescued the delay-of-cell-death defect of the ced-8(n1891) mutant and restored wild-type cell corpse patterns to the ced-8(n1891) embryos ( Fig. 1e ), indicating that Asp 163 is not important for CED-8’s proapoptotic function. By contrast, P ced-8 CED-8(D21A)::GFP did not rescue the delay-of-cell-death defect of the ced-8(n1891) mutant ( Fig. 1f ), although the GFP intensity on the plasma membrane of P ced-8 CED-8(D21A)::GFP transgenic embryos was similar to that of P ced-8 CED-8::GFP or P ced-8 CED-8(D163A)::GFP embryos ( Supplementary Fig. S2 ). This result indicates that CED-3 cleavage at the Asp 21 site is critical for CED-8’s proapoptotic function in vivo . Finally, expression of the carboxy-terminal cleavage fragment of CED-8 by CED-3 [P ced-8 CED-8(22–458)::GFP] also fully rescued the ced-8(n1891) mutant ( Fig. 1f ), indicating that CED-8(22–458), which we named acCED-8, is sufficient to mediate the proapoptotic function of CED-8 and represents the CED-3-activated form of CED-8. CED-8 is crucial for PS externalization in apoptotic cells To probe how ced-8 regulates apoptosis, we examined whether ced-8 affects the PS externalization process, a hallmark of apoptosis [1] , [2] , [7] , and one of the earliest detectable cell death events in C. elegans [14] . We used a genetically encoded PS sensor, secreted Annexin V::GFP fusion (ANV::GFP) [14] , to monitor the PS externalization process. In early comma-stage wild-type C. elegans embryos carrying an integrated transgene smIs76 , which expresses ANV::GFP under the control of the C. elegans heat-shock promoters [14] , an average of nine cell corpses were observed ( Fig. 1a ) and almost all of them were strongly labelled by ANV::GFP ( Fig. 2a,d ). In comma-stage smIs76; ced-8(n1891) embryos, only a few cell corpses were observed and ~60% of them were labelled by ANV::GFP ( Figs 1a and 2b–d ). However, in those apoptotic cells that were labelled, ANV::GFP labelling often was weak or barely detectable ( Fig. 2c,e ), with an average fluorescent intensity ~11% of that seen in apoptotic cells in wild-type embryos ( Fig. 2e ). These results indicate that loss of ced-8 blocks or greatly reduces PS externalization in cells that already died at this stage. As the death of most cells programmed to die at the comma stage was deferred to later embryonic stages, we examined whether apoptotic cells observed in late-stage ced-8(n1891) embryos were labelled by ANV::GFP. In 4-fold ced-8(n1891) embryos, there are an average of 15 cell corpses compared with an average of 0.5 cell corpse in wild-type 4-fold embryos ( Fig. 1a ). However, only 5% of these apoptotic cells in smIs76; ced-8(n1891) 4-fold embryos were labelled by ANV::GFP ( Fig. 2d ), indicating that PS was not externalized in cells that died in late-stage ced-8(n1891) embryos either. We obtained similar results using another genetically encoded PS sensor, secreted GFP::Lactadherin fusion (GFP::Lact) [14] . In smIs434 animals, which carry an integrated transgene expressing GFP::Lact under the control of the heat-shock promoters [14] , ced-8(n1891) not only reduced the percentage of apoptotic cells labelled by GFP::Lact ( Supplementary Fig. S3a ) but also markedly decreased the intensity of GFP::Lact labelling on apoptotic cells ( Supplementary Fig. S3b ), providing further evidence that loss of ced-8 greatly reduces PS externalization in apoptotic cells. 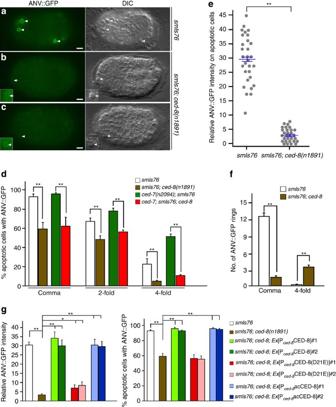Figure 2: PS externalization in apoptotic cells is blocked or greatly reduced in theced-8mutant. (a–c) ANV::GFP and differential contrast interference images of comma-stage embryos fromsmIs76andsmIs76; ced-8(n1891)animals are shown. Arrowheads indicate apoptotic cells labelled by ANV::GFP. InsmIs76; ced-8(n1891)embryos, apoptotic cells were either not labelled (indicated by an arrow,b) or were very weakly labelled (c) by ANV::GFP. Insets show enhanced GFP images of apoptotic cells. Scale bars, 5 μm. (d) Percentages of apoptotic cells labelled by ANV::GFP in the indicated strains and stages are shown. (e) Relative intensity of ANV::GFP that labelled apoptotic cells in comma-stage embryos was quantified in the indicated strains (see Methods). Results are shown using the histogram (n=30), with mean±s.e.m. indicated. Apoptotic cells that were not labelled by ANV::GFP are presented with zero intensity. (f) The number of ANV::GFP rings in the indicated strains was scored in the comma- and 4-fold-stage embryos regardless of their cell morphology. (g) Rescue of the PS externalization defect of theced-8(n1891)mutant by variousced-8transgenes. Quantification of the percentage of apoptotic cells labelled by ANV::GFP and the relative intensity of ANV::GFP in transgenic embryos was performed as indande. (d,f,g) Results are presented as mean±s.e.m. (n=15 each). The significance of differences between results was determined by two-tailed Student’st-tests, *P<0.05; **P<0.001. Heat-shock treatment was performed at 33°C for 30 min and embryos were examined after 2 h recovery at 20 °C. Exposure time for each fluorescent image was identical (12.5 ms). Figure 2: PS externalization in apoptotic cells is blocked or greatly reduced in the ced-8 mutant. ( a – c ) ANV::GFP and differential contrast interference images of comma-stage embryos from smIs76 and smIs76; ced-8(n1891) animals are shown. Arrowheads indicate apoptotic cells labelled by ANV::GFP. In smIs76; ced-8(n1891) embryos, apoptotic cells were either not labelled (indicated by an arrow, b ) or were very weakly labelled ( c ) by ANV::GFP. Insets show enhanced GFP images of apoptotic cells. Scale bars, 5 μm. ( d ) Percentages of apoptotic cells labelled by ANV::GFP in the indicated strains and stages are shown. ( e ) Relative intensity of ANV::GFP that labelled apoptotic cells in comma-stage embryos was quantified in the indicated strains (see Methods). Results are shown using the histogram ( n =30), with mean±s.e.m. indicated. Apoptotic cells that were not labelled by ANV::GFP are presented with zero intensity. ( f ) The number of ANV::GFP rings in the indicated strains was scored in the comma- and 4-fold-stage embryos regardless of their cell morphology. ( g ) Rescue of the PS externalization defect of the ced-8(n1891) mutant by various ced-8 transgenes. Quantification of the percentage of apoptotic cells labelled by ANV::GFP and the relative intensity of ANV::GFP in transgenic embryos was performed as in d and e . ( d , f , g ) Results are presented as mean±s.e.m. ( n =15 each). The significance of differences between results was determined by two-tailed Student’s t -tests, * P <0.05; ** P <0.001. Heat-shock treatment was performed at 33°C for 30 min and embryos were examined after 2 h recovery at 20 °C. Exposure time for each fluorescent image was identical (12.5 ms). Full size image We then performed time-lapse microscopy to follow the PS externalization process in cells undergoing apoptosis. As reported previously [14] , in wild-type C. elegans embryos, ANV::GFP was detected on the surface of the dying cell before it adopted the typical button-like cell corpse morphology ( Supplementary Fig. S4a,b ). The intensity of ANV::GFP increased as the dying cell shrank and displayed the dense button-like morphology ( Supplementary Fig. S4c ), and reached its maximum around the time when it was engulfed by one of its neighbours ( Supplementary Fig. S4d ), which were also weakly labelled by ANV::GFP [14] . In the ced-8(n1891) embryo, ANV::GFP labelling of the apoptotic cell was much weaker ( Supplementary Fig. S4h–n ) and was first detected after the dying cell already adopted the button-like morphology ( Supplementary Fig. S4h,i ), the appearance of which was delayed compared with that in wild-type embryos (20 versus 10 min in the N2 embryo; Supplementary Fig. S4c,i ). The intensity of ANV::GFP on the apoptotic cell did not increase subsequently and the apoptotic cell persisted for a significantly longer time period (120 versus 30 min in the N2 embryo; Supplementary Fig. S4c–g, i–n ), which suggests a potential defect in cell corpse engulfment (see below). The observations from the time-lapse microscopy provide further support that ced-8 has a critical role in PS externalization in apoptotic cells. It is possible that in ced-8(n1891) animals, the cells programmed to die in early embryonic stages already initiated the suicide programme and exposed PS, but had not yet adopted the button-like morphology. We thus quantified the total number of ANV::GFP rings in comma-stage embryos regardless of their morphology and found that wild-type embryos had an average of 12 ANV::GFP rings, most of which displayed apoptotic cell morphology ( Fig. 2f ). By contrast, ced-8(n1891) comma-stage embryos had an average of 1.5 ANV::GFP rings ( Fig. 2f ), confirming that most cells programmed to die at the comma stage did not expose PS at this stage. We further sensitized quantification of PS exposure in apoptotic cells by inactivating the ced-7 gene, which encodes an ATP-binding cassette transporter important for cell corpse engulfment [24] and promotes time-dependent efflux of exposed PS from the surface of apoptotic cells to the extracellular space through PS-containing small vesicles [14] , [25] . Loss of ced-7 leads to retention of exposed PS on the surface of aged or unengulfed apoptotic cells and thus sensitizes scoring of apoptotic cells with surface-exposed PS. In comma-stage ced-7(n2094) embryos, almost all apoptotic cells (97%) were labelled by ANV::GFP, whereas in 4-fold ced-7(n2094) embryos, 52% of unengulfed cell corpses still had surface-exposed PS ( Fig. 2d ). In comparison, only 6% of unengulfed cell corpses in ced-1(e1735) 4-fold embryos have surface-exposed PS because of efflux and loss of exposed PS from apoptotic cells [14] . In ced-7(n2094); ced-8(n1891) embryos, 63% of cell corpses in the comma stage were labelled by ANV::GFP and only 11% of unengulfed cell corpses were labelled by ANV::GFP in late 4-fold embryos ( Fig. 2d ), which had the same number of unengulfed apoptotic cells as that in ced-7(n2094) 4-fold embryos ( Fig. 4c ). These observations confirm that loss of ced-8 also significantly reduces PS exposure in unengulfed apoptotic cells. Taken together, these results indicate that ced-8 is crucial for PS externalization in apoptotic cells. Figure 4: ced-8 is important for cell corpse engulfment in C. elegans . 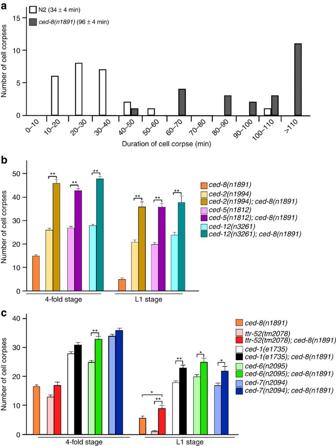Figure 4:ced-8is important for cell corpse engulfment inC. elegans. (a) Time-lapse microscopy analysis of the durations of cell corpses. The persistence of 25 cell corpses from N2 embryos (n=3) and 24 cell corpses fromced-8(n1891)embryos (n=8) was monitored. The numbers in parentheses indicate the average persistence for cell corpses±s.e.m. They-axis indicates the number of cell corpses with a specific duration range (shown by thex-axis). The durations of four cell divisions in the MS cell lineage from the MS cell to the MS.aaaa cell38were also followed to ensure that the embryos assayed had similar rates of development. The average duration of four cell divisions for N2 embryos is 89±6 and 91±3 min forced-8(n1891)embryos. (b,c) Theced-8(n1891)mutation enhances the corpse clearance defect of engulfment mutants. Cell corpses were scored in 4-fold embryos and in L1 larvae from the indicated strains. They-axis represents the mean of cell corpses scored in the whole embryos or in the head region of L1 larvae (n=15). Error bar represents s.e.m. The significance of differences between results was determined by two-tailed Student’st-tests, *P<0.05; **P<0.001. ( a ) Time-lapse microscopy analysis of the durations of cell corpses. The persistence of 25 cell corpses from N2 embryos ( n =3) and 24 cell corpses from ced-8(n1891) embryos ( n =8) was monitored. The numbers in parentheses indicate the average persistence for cell corpses±s.e.m. The y -axis indicates the number of cell corpses with a specific duration range (shown by the x -axis). The durations of four cell divisions in the MS cell lineage from the MS cell to the MS.aaaa cell [38] were also followed to ensure that the embryos assayed had similar rates of development. The average duration of four cell divisions for N2 embryos is 89±6 and 91±3 min for ced-8(n1891) embryos. ( b , c ) The ced-8(n1891) mutation enhances the corpse clearance defect of engulfment mutants. Cell corpses were scored in 4-fold embryos and in L1 larvae from the indicated strains. The y -axis represents the mean of cell corpses scored in the whole embryos or in the head region of L1 larvae ( n =15). Error bar represents s.e.m. The significance of differences between results was determined by two-tailed Student’s t -tests, * P <0.05; ** P <0.001. Full size image CED-8 is activated by CED-3 to promote PS externalization We next examined whether CED-3 cleavage of CED-8 at the Asp 21 site is critical for CED-8 to promote PS externalization in apoptotic cells. Transgenes expressing wild-type or altered forms of CED-8 under the control of the ced-8 gene promoter were introduced into smIs76; ced-8(n1891) animals. The percentage of apoptotic cells labelled by ANV::GFP and the intensity of ANV::GFP labelling in comma-stage transgenic embryos were examined ( Fig. 2g ). Expression of wild-type CED-8 or acCED-8 in smIs76; ced-8(n1891) embryos restored ANV::GFP labelling of apoptotic cells to the levels seen in smIs76 embryos ( Fig. 2g ), indicating full rescue of the PS externalization defect. By contrast, ANV::GFP labelling of apoptotic cells in smIs76; ced-8(n1891) embryos expressing CED-8(D21E) was similar to that seen in smIs76; ced-8(n1891) embryos ( Fig. 2g ), indicating no rescue of the PS externalization defect. These results indicate that CED-3 cleavage at the Asp 21 site is also critical for activating CED-8’s function in promoting PS externalization in apoptotic cells. Given that acCED-8 is necessary and sufficient to mediate the PS externalization activity of CED-8 in apoptotic cells, we examined whether acCED-8 can induce PS exposure in non-apoptotic cells. We induced global expression of acCED-8 under the control of the C. elegans heat-shock promoters (P hsp acCED-8) and then examined PS exposure using GFP::Lact, which is more sensitive in detecting PS exposure in living cells than ANV::GFP ( Supplementary Fig. S5 ) [14] , [26] . In smIs434 animals expressing GFP::Lact, GFP::Lact only labelled apoptotic cells (arrowheads, Fig. 3a ). Expression of acCED-8 in smIs434 embryos resulted in GFP::Lact labelling of all cells, including both living cells and apoptotic cells ( Fig. 3c ), suggesting that acCED-8 can induce ectopic PS exposure on the surface of all cells. In comparison, expression of full-length CED-8 (P hsp CED-8) in smIs434 embryos did not alter the staining pattern of GFP::Lact or cause widespread, ectopic PS exposure on the surface of all cells ( Fig. 3b ). In ced-3(n2433); smIs434 animals, where almost all apoptosis is blocked, expression of acCED-8, but not full-length CED-8, still caused all cells to externalize PS ( Fig. 3d,e ), indicating that acCED-8 is capable of activating PS externalization independent of the CED-3 caspase and apoptosis. 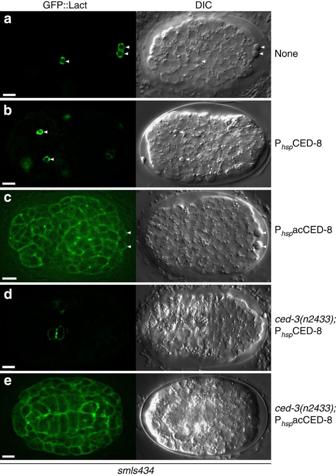These results suggest that CED-8, once activated by CED-3, promotes PS externalization in cells through the generation of acCED-8. Figure 3: Expression of acCED-8 induces ectopic PS exposure in all cells. (a–e) GFP::Lact and differential contrast interference images of comma-stage embryos from the following strains are shown:smIs434(a),smIs434; ex[PhspCED-8] (b),smIs434; ex[PhspacCED-8] (c),ced-3(n2433); smIs434; ex[PhspCED-8] (d) andced-3(n2433); smIs434; ex[PhspacCED-8] (e). Arrowheads indicate apoptotic cells. Heat-shock treatment was performed at 33°C for 45 min and embryos were examined after 2 h recovery at 20 °C. Exposure time for each fluorescent image was identical (100 ms). Scale bars, 5 μm. Figure 3: Expression of acCED-8 induces ectopic PS exposure in all cells. ( a – e ) GFP::Lact and differential contrast interference images of comma-stage embryos from the following strains are shown: smIs434 ( a ), smIs434; ex [P hsp CED-8] ( b ), smIs434; ex [P hsp acCED-8] ( c ), ced-3(n2433); smIs434; ex [P hsp CED-8] ( d ) and ced-3(n2433); smIs434; ex [P hsp acCED-8] ( e ). Arrowheads indicate apoptotic cells. Heat-shock treatment was performed at 33°C for 45 min and embryos were examined after 2 h recovery at 20 °C. Exposure time for each fluorescent image was identical (100 ms). Scale bars, 5 μm. Full size image CED-8 is important for cell corpse engulfment As surface-exposed PS is an important ‘eat-me’ signal for phagocytosis [2] , [4] , [27] and because cell corpses in ced-8(n1891) embryos appear to persist significantly longer than those in wild-type embryos ( Supplementary Fig. S4 ), we investigated whether ced-8 affects cell corpse engulfment in C. elegans, in addition to its previously reported role in regulating the kinetics of cell death [15] . We first used four-dimensional microscopy to measure the duration of embryonic cell corpses in ced-8(n1891) animals [28] . In wild-type embryos, on average cell corpses persisted for 34 min. In ced-8(n1891) embryos, cell corpses persisted for 96 min, which is almost three times longer than that of wild-type animals ( Fig. 4a ). These results indicate that the cell corpse engulfment process is significantly compromised in the ced-8(n1891) mutant. In C. elegans, two partially redundant pathways mediate cell corpse removal, with ced-1, ced-6, ced-7 and ttr-52 genes functioning in one pathway and ced-2, ced-5 and ced-12 genes acting in the other [29] , [30] , [31] . To interrogate the functioning pathway of ced-8 , we constructed and analysed double mutants between the ced-8(n1891) mutation and strong lf alleles of the above engulfment genes. ced-8(n1891) markedly enhanced the cell corpse engulfment defect of the ced-2, ced-5 or ced-12 mutants at the late 4-fold embryonic stage and L1 larval stage ( Fig. 4b ), but only mildly enhanced the corpse engulfment defect of the ced-1, ced-6, ced-7 or ttr-52 mutants at the L1 larval stage ( Fig. 4c ). These results are consistent with ced-8 acting to promote PS externalization, which serves as an ‘eat-me’ signal for both cell corpse engulfment pathways to promote phagocytosis of apoptotic cells ( Fig. 5 ) [26] , [28] , [31] . 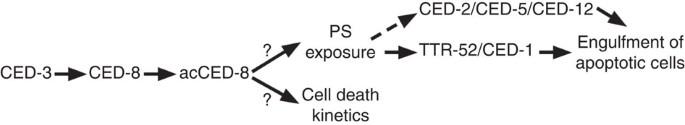Figure 5: CED-8 working model. CED-8 is cleaved and activated by CED-3 during apoptosis to generate acCED-8, which promotes PS externalization and normal progression of apoptosis through undefined mechanisms (?). Surface-exposed PS then promotes phagocytosis of apoptotic cells through TTR-52, a PS-binding extracellular bridging molecule, and its binding partner, the CED-1 phagocyte receptor. Surface-exposed PS may also promote phagocytosis of apoptotic cells through the CED-2/CED-5/CED-12 engulfment pathway. Figure 5: CED-8 working model. CED-8 is cleaved and activated by CED-3 during apoptosis to generate acCED-8, which promotes PS externalization and normal progression of apoptosis through undefined mechanisms (?). Surface-exposed PS then promotes phagocytosis of apoptotic cells through TTR-52, a PS-binding extracellular bridging molecule, and its binding partner, the CED-1 phagocyte receptor. Surface-exposed PS may also promote phagocytosis of apoptotic cells through the CED-2/CED-5/CED-12 engulfment pathway. Full size image As a multipass plasma membrane protein, how CED-8 affects programmed cell death has been a major unresolved issue in C. elegans apoptosis. In this study, we demonstrate that CED-8 acts downstream of the CED-3 caspase to promote apoptosis and is a substrate of CED-3. Cleavage of CED-8 by CED-3 is required to activate CED-8’s proapoptotic functions and generates a C-terminal cleavage product, acCED-8, that is sufficient to mediate the proapoptotic functions of CED-8. Importantly, ced-8 is also critical for PS externalization in apoptotic cells, which is an unexpected new role for CED-8. Cleavage of CED-8 by CED-3 is also required to activate its PS externalization activity. Moreover, ectopic expression of acCED-8, but not full-length CED-8, can induce PS externalization in all living cells in the absence of the CED-3 caspase or apoptosis. Our study thus identifies a crucial link between caspase activation and PS externalization [4] , [27] . Consistent with its role in promoting PS externalization in apoptotic cells, we find that ced-8 is important for cell corpse engulfment. Loss of ced-8 causes persistence of embryonic cell corpses, mildly enhances the cell corpse engulfment defects of ced-1, ced-6, ced-7 and ttr-52 mutants and strongly enhances the cell corpse engulfment defects of ced-2, ced-5 and ced-12 mutants. As PS could be an ‘eat-me’ signal for both cell corpse engulfment pathways in C. elegans [26] , [28] , [31] , our observations are consistent with ced-8 acting in both engulfment pathways to promote clearance of apoptotic cells ( Fig. 5 ). However, given the significantly stronger effect of ced-8(n1891) in enhancing the engulfment defect of the ced-2 pathway and marginal effect in enhancing the engulfment defect of the ced-1 pathway, ced-8 may mainly act through the ced-1, ced-6, ced-7 and ttr-52 engulfment pathway to promote phagocytosis. As ced-1 encodes a phagocyte receptor that recognizes and promotes engulfment of apoptotic cells with surface-exposed PS through its binding partner TTR-52, a PS-binding extracellular bridging protein [31] , [32] , our finding delineates a new apoptotic signalling cascade, starting from CED-3 caspase activation during apoptosis, followed by CED-3-mediated activation of CED-8, acCED-8-mediated activation of PS exposure on the surface of apoptotic cells, and subsequent recognition and removal of PS-exposed apoptotic cells by the TTR-52 and CED-1 phagocytosis pathway, which is probably aided by the ced-2, ced-5 and ced-12 phagocytosis pathway, also capable of recognizing and engulfing apoptotic cells with surface-exposed PS ( Fig. 5 ). A new study reports a similar finding that a mammalian XK family protein, Xkr8, and its C. elegans homologue CED-8 have a conserved role in promoting PS exposure in apoptotic cells [33] . The PS-externalizing activity of Xkr8 also appears to be activated by caspase cleavage. Interestingly, CED-8 is cleaved and activated by the CED-3 caspase at the N terminus, whereas Xkr8 is cleaved and potentially activated by mammalian caspases at its C terminus ( Supplementary Fig. S6 ). Although the activated form of Xrk8 has not been identified [33] , the N-terminal cleavage product of Xrk8 shares an overall sequence similarity to acCED-8, including all putative transmembrane domains. Moreover, the 21-residue CED-8 N-terminal sequence removed by CED-3 cleavage seems to be unique to C. elegans and is not found in Xkr8 or Xkr8 homologues in other organisms. It remains to be determined whether CED-8 and Xkr8 are regulated by similar factors and activated through a conserved mechanism, and whether activated CED-8 and activated Xkr8 promote PS externalization in apoptotic cells through a similar mechanism. CED-8 shares sequence similarity to the XK transporters. However, the substrates that XK family proteins might transport remain unknown [18] , [33] . Given our new findings, it is conceivable that acCED-8 may directly transport PS across the plasma membrane to effect PS exposure. However, because CED-8 also affects the kinetics of apoptosis, it is more likely that acCED-8 is a general caspase mediator that interacts with several downstream effectors to promote cell death execution ( Fig. 5 ). In this scenario, acCED-8 may regulate the activity of a lipid-transporting enzyme, leading to PS externalization in apoptotic cells. Moreover, because loss of ced-8 does not completely abolish PS externalization in C. elegans apoptotic cells, additional mechanisms or regulators must be responsible for the residual PS externalization activity in the ced-8 mutant during apoptosis. Strains and culture conditions C. elegans strains were maintained using standard procedures [34] . The following alleles were used in the genetic analyses: LGI, ced-1(e1735), ced-12(n3261), smIs111 ; LGIII, ced-6(n2095), ced-7(n2094), ttr-52(tm2078) ; LGIV, ced-2(n1994), ced-3(n2433), ced-5(n1812) ; LGV, smIs76 ; and LGX, ced-8(n1891), smIs434 . smIs76 and smIs434 are integrated transgenes generated by ultraviolet irradiation of animals carrying extrachromosomal arrays containing P hsp ANV::GFP and P hsp GFP::Lact, respectively [14] . They were backcrossed four times with wild-type animals before being used for genetic analyses. Transgenic animals Transgenic animals were generated using standard protocols [35] . P ced-8 CED-8::GFP, P ced-8 CED-8(D21A)::GFP, P ced-8 CED-8(D163A)::GFP or P ced-8 acCED-8::GFP was injected into unc-76(e911); ced-8(n1891) animals at 5 ng μl −1 along with an unc-76 rescuing plasmid (at 50 ng μl −1 ) as a co-injection marker. P ced-8 CFP::CED-8 and P ced-8 YFP::CED-8(D21E) were co-injected into ced-1(e1375); unc-76(e911) animals at 25 ng μl −1 each along with the unc-76 rescuing plasmid (at 50 ng μl −1 ). P hsp CED-8 or P hsp acCED-8 was injected into smIs434 or ced-3(n2433); smIs434 animals at 25 ng μl −1 along with the P sur-5 mCherry plasmid (25 ng μl −1 ) as a co-injection marker, which directs mCherry expression in all somatic cells in most developmental stages [36] . Quantification of cell corpses The number of cell corpses in living embryos or in the head region of L1 larvae was scored using Nomarski optics [37] . Quantification of ANV::GFP or GFP::Lact intensity on corpses To score the number of cell corpses labelled by ANV::GFP or GFP::Lact, apoptotic cells were first identified using differential contrast interference optics and then examined for the presence of ANV::GFP or GFP::Lact on their surface. To measure the ANV::GFP or GFP::Lact fluorescence intensity on cell corpses, fluorescence micrographs were captured using a Zeiss Axioplan 2 microscope (Zeiss) equipped with a charge-coupled device camera and the Slidebook 5.0 software (Intelligent Imaging Innovations). GFP intensity was determined by measuring the fluorescence signals from three random areas on the plasma membrane of each apoptotic cell (Ia) and three random areas on normal cells (Ib). The average value of Ia minus the average value of Ib was then used as the value for relative ANV::GFP or GFP::Lact intensity. Quantification of ANV::GFP rings C. elegans embryos were mounted on slides using the egg salt buffer (118 mM NaCl, 48 mM KCl, 2 mM CaCl 2 , 2 mM MgCl 2 , 5 mM HEPES pH 7.5) and the number of ANV::GFP rings was then scored regardless of the cell morphology. Heat-shock treatment For time-lapse microscopy, smIs76 or smIs76; ced-8(n1891) embryos were placed at 33°C for 30 min, followed by recovery at room temperature for 1 h. For analysis of ANV::GFP or GFP::Lact labelling of comma-stage embryos, embryos were placed at 33°C for 45 min, followed by recovery at room temperature 2 h. For analysis of ANV::GFP or GFP::Lact labelling of 4-fold-stage embryos, embryos were placed at 33°C for 45 min, followed by recovery at room temperature for 3 h. Microscopy For fluorescent microscopy, C. elegans embryos were mounted on agar pads and observed using × 100 optics on Axioplan 2 microscopes (Zeiss). Fluorescence and differential contrast interference images were captured using a charge-coupled device camera (PCO SensiCam) coupled with the Slidebook 5.0 software. To perform time-lapse microscopy, C. elegans embryos were mounted on slides with agar pad in egg salt buffer and cover slips were sealed with Beeswax and Vaseline (1:1). Images in a 45-micron z-series (3 micron per section) were captured every 2 or 5 min for 180–360 min. Neutral density filter was used to allow only 12% light transmission. Four-dimensional microscopy analysis of cell corpse durations in the N2 and ced-8(n1891) embryos were performed as described previously [28] . Molecular biology ced-8- coding region was amplified using PCR from the pBluescript KS(+)- ced-8 vector [15] and subcloned into the pET-41b vector (Novagen) through its Spe I and Eco RV sites. Deletions of CED-8 or single amino-acid substitutions in CED-8 were generated by site-directed mutagenesis of the resulting pET-41b-CED-8 vector. The P ced-8 CED-8::GFP vector was made by fusing a 1.2-kb ( Sma I/ Nhe I) ced-8 prompter to a ced-8 cDNA ( Nhe I/ Age I) in frame with GFP from pPD95.77. The P ced-8 CFP::CED-8 and P ced-8 YFP::CED-8(D21E) vectors were made by fusing the 1.2 kb ced-8 promoter to CFP::CED-8 and YFP::CED-8(D21E), respectively. P hsp acCED-8 was made by PCR amplification of ced-8 cDNA encoding amino acids 22–458 and subcloning the PCR fragment into the pPD49.78 and pPD49.83 vectors through Nhe I and Eco R V sites. CED-3 protease assays CED-3 protease assays were carried out using the standard protocol [22] . Briefly, GST-CED-8, GST-CED-8(D21A), GST-CED-8(D21E), GST-CED-8(D163A) and GST-CED-8(D21A, D163A) were synthesized and labelled with 35 S -methionine using TNT Transcription/Translation coupled system (Promega) and incubated with 5 ng of purified CED-3 at 30 °C for 2 h. The reactions were then resolved by 15% SDS–PAGE. Statistical analysis P -values represent analysis from two-tailed Student’s t -tests. * P <0.05; ** P <0.001. How to cite this article: Chen, Y.-Z. et al. Caspase-mediated activation of Caenorhabditis elegans CED-8 promotes apoptosis and phosphatidylserine externalization. Nat. Commun. 4:2726 doi: 10.1038/ncomms3726 (2013).